Revealing the high-energy electronic excitations underlying the onset of high-temperature superconductivity in cuprates In strongly correlated systems the electronic properties at the Fermi energy ( E F ) are intertwined with those at high-energy scales. One of the pivotal challenges in the field of high-temperature superconductivity (HTSC) is to understand whether and how the high-energy scale physics associated with Mott-like excitations (| E − E F |>1 eV) is involved in the condensate formation. Here, we report the interplay between the many-body high-energy CuO 2 excitations at 1.5 and 2 eV, and the onset of HTSC. This is revealed by a novel optical pump-supercontinuum-probe technique that provides access to the dynamics of the dielectric function in Bi 2 Sr 2 Ca 0.92 Y 0.08 Cu 2 O 8+ δ over an extended energy range, after the photoinduced suppression of the superconducting pairing. These results unveil an unconventional mechanism at the base of HTSC both below and above the optimal hole concentration required to attain the maximum critical temperature ( T c ). The high- T c copper-oxide (cuprate) superconductors are a particular class of strongly correlated systems in which the interplay [1] between the Cu-3 d and the O-2 p states determines both the electronic structure close to the Fermi level as well as the high-energy properties related to the formation of Zhang–Rice singlets [2] (hole shared among the four oxygen sites surrounding a Cu, and antiferromagnetically coupled to the Cu spin; energy E ZR ∼ 0.5 eV) and to the charge-transfer processes [3] ( Δ CT ∼ 2 eV). One of the unsolved issues of high- T c superconductivity is whether and how the electronic many-body excitations at high-energy scales are involved in the condensate formation in the under- and over-doped regions of the superconducting dome. Solving this problem would provide a benchmark for unconventional models of high- T c superconductivity, at variance with the BCS theory of conventional superconductivity, where the opening of the superconducting gap induces a significant rearrangement of the quasiparticle excitation spectrum over an energy range of only a few times 2 Δ SC (ref. 4 ). As the knowledge of the dielectric function ɛ ( ω ) provides direct information about the underlying electronic structure, optical spectroscopic techniques have been widely used to investigate high- T c superconductors [5] , [6] , [7] , [8] , [9] , [10] , [11] , [12] , [13] , [14] , [15] , [16] , [17] . Recently, equilibrium techniques revealed a superconductivity-induced modification of the CuO 2 -planes' optical properties involving energy scales in excess of 1 eV (refs 7 , 11 , 12 , 14 , 15 , 16 , 17 ). These results suggested a possible superconductivity-induced gain in the in-plane kinetic-energy on the underdoped side of the phase diagram [18] , [19] , [20] . However, the identification of the high-energy electronic excitations involved in the onset of high-temperature superconductivity (HTSC) has remained elusive because they overlap in energy with the temperature-dependent narrowing of the Drude-like peak. Here we solve this question adopting a non-equilibrium approach to disentangle the ultrafast modifications of the high-energy spectral weight ( , σ 1 ( ω )= ɛ 2 ( ω )· ω /4 πi being the real part of the optical conductivity) from the slower broadening of the Drude-like peak induced by the complete electron-boson thermalization. As the superconducting gap (2 Δ SC ) value is related to the total number of excitations [21] , an impulsive suppression [22] of 2 Δ SC is achieved by photoinjecting excess quasiparticles in the superconducting Bi 2 Sr 2 Ca 0.92 Y 0.08 Cu 2 O 8+ δ crystals (Y-Bi2212), through an ultrashort light pulse (pump). Exploiting the supercontinuum spectrum produced by a nonlinear photonic crystal fibre [23] we are able to probe the high-energy (1.2–2.2 eV) modifications of the ab -plane optical properties at low pump fluences (<10 μJ cm −2 ), avoiding the complete vaporization of the superconducting phase [22] , [24] . This novel time-resolved optical spectroscopy (Methods) allows us to demonstrate the interplay between many-body electronic excitations at 1.5 and 2 eV and the onset of superconductivity both below and above the optimal hole concentration required to attain the maximum T c . Equilibrium optical properties of Bi 2 Sr 2 Ca 0.92 Y 0.08 Cu 2 O 8+ δ The interpretation of time-resolved optical spectroscopy relies on the detailed knowledge of the equilibrium (intragap transitions) ɛ ( ω ) of the system. 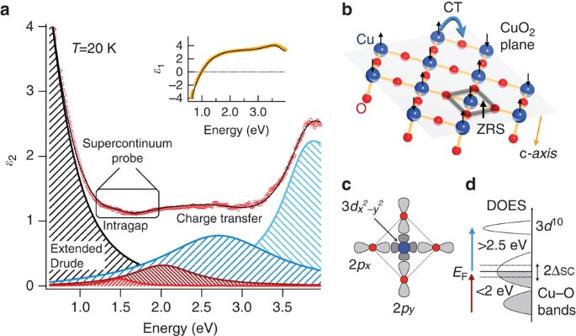Figure 1: Dielectric function of optimally doped Bi2Sr2Ca0.92Y0.08Cu2O8+δ. (a) The high-energy region of the imaginary part of theab-plane dielectric function, measured atT=20 K for the optimally doped sample (estimated hole concentrationp=0.16, ref.46), is shown. The thin black line is the fit to the data described in the text. The values of the parameters resulting from the fit are reported in theSupplementary Table S1. The contributions of the individual interband oscillators atω0i∼1.46, 2, 2.72 and 3.85 eV are indicated as colour-patterned areas. The real part of the dielectric function, with the respective fit, is shown in the inset.Supplementary Figure S1shows the fits to the reflectivity forT=300 and 100 K and the extractedI2χ(Ω). (b) Schematics of the ZRS and of the in-plane CT process between Cu and O atoms. (c) The atomic orbitals involved in the charge transfer and Zhang-Rice singlet (ZRS) are schematically indicated. (d) Cartoon of the electron density of states (DOES) (ref.27). The red and blue arrows represent transitions between mixed Cu–O states and involving a 3d10configuration in the final state, respectively. In Figure 1a , we report the real ( ɛ 1 ) and imaginary ( ɛ 2 ) parts of the dielectric function, measured on an optimally doped sample ( T c =96 K, labelled OP96) by spectroscopic ellipsometry at 20 K (Methods). Below 1.25 eV, ɛ ( ω ) is dominated by the Drude response of free carriers coupled to a broad spectrum of bosons I 2 χ ( Ω ) (refs 25 , 26 ). In the high-energy region ( ℏ ω >1.25 eV), the interband transitions dominate. The best fit to the data (solid black lines) is obtained by modelling the equilibrium dielectric function as a sum of an extended Drude term ( ɛ D ) and Lorentz oscillators at 0.5 eV and higher energies ( ɛ L , indexed by i ): ɛ eq ( T , ω )= ɛ D ( T , ω )+Σ i ɛ L i ( T , ω ) ( Supplementary Note 1 ). The high-energy region of ɛ ( ω ) is characterized by interband transitions at ω 0 i ∼ 1.46, 2, 2.72 and 3.85 eV. The attribution of the interband transitions in cuprates is a subject of intense debate. As a general phenomenological trend, the charge-transfer (CT) gap edge (hole from the upper Hubbard band with d x 2 - y 2 symmetry to the O-2 p x,y orbitals, Fig. 1b,c ) in the undoped compounds is about 2 eV (ref. 5 ). Upon doping, a structure reminiscent of the CT gap moves to higher energies, while the gap is filled with states (intragap transitions) at the expense of spectral weight at ℏ ω >2 eV (ref. 5 , Fig. 1d ). Dynamical mean field calculations of the electron spectral function and of the ab -plane optical conductivity for the hole-doped three-band Hubbard model recently found that the Fermi level moves into a broad ( ∼ 2 eV) and structured band of mixed Cu–O character, corresponding to the Zhang–Rice singlet states [27] . The empty upper Hubbard band, which involves Cu–3 d [10] states, is shifted to higher energies with respect to the undoped compound, accounting for the blue shift of the optical CT edge to 2.5–3 eV. The structures appearing in the optical conductivity at 1–2 eV, that is, below the remnant of the CT gap, are mostly related to transitions between many-body Cu–O states at binding energies as high as 2 eV (for example singlet states) and states at the Fermi energy. Figure 1: Dielectric function of optimally doped Bi 2 Sr 2 Ca 0.92 Y 0.08 Cu 2 O 8+ δ . ( a ) The high-energy region of the imaginary part of the ab -plane dielectric function, measured at T =20 K for the optimally doped sample (estimated hole concentration p =0.16, ref. 46 ), is shown. The thin black line is the fit to the data described in the text. The values of the parameters resulting from the fit are reported in the Supplementary Table S1 . The contributions of the individual interband oscillators at ω 0i ∼ 1.46, 2, 2.72 and 3.85 eV are indicated as colour-patterned areas. The real part of the dielectric function, with the respective fit, is shown in the inset. Supplementary Figure S1 shows the fits to the reflectivity for T =300 and 100 K and the extracted I 2 χ (Ω). ( b ) Schematics of the ZRS and of the in-plane CT process between Cu and O atoms. ( c ) The atomic orbitals involved in the charge transfer and Zhang-Rice singlet (ZRS) are schematically indicated. ( d ) Cartoon of the electron density of states (DOES) (ref. 27 ). The red and blue arrows represent transitions between mixed Cu–O states and involving a 3 d 10 configuration in the final state, respectively. 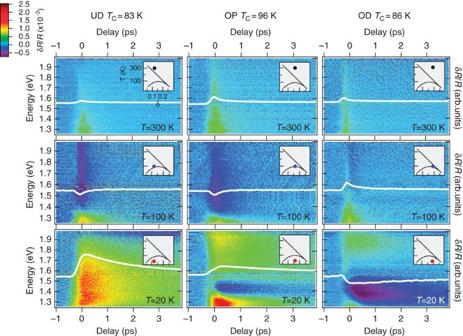Figure 2: Energy- and time-resolved reflectivity on Bi2Sr2Ca0.92Y0.08Cu2O8+δ. The dynamics of the reflectivity is measured over a broad spectral range. The two-dimensional scans of δR/R(ω,t) are reported for three different doping regimes (first column: underdoped (UD),Tc=83 K; second column: optimally doped (OP),Tc=96 K; third column: overdoped (OD),Tc=86 K), in the normal (first row), pseudogap (second row) and superconducting phases (third row). See Methods for estimation of hole contentp. The insets display schematically the position of each scan in theT-pphase diagram of Bi2Sr2Ca0.92Y0.08Cu2O8+δ. The white lines (right axes) are the time traces at 1.5 eV photon energy. Full size image Time-resolved optical spectroscopy In Figure 2, we report the time- and frequency-resolved reflectivity variation in the 1.2–2 eV spectral range (δ R/R ( ω , t )= R neq ( ω , t )/ R eq ( ω , t )-1, where R neq ( ω , t ) and R eq ( ω , t ) are the non-equilibrium (pumped) and equilibrium (unpumped) reflectivities), for the normal (top row), pseudogap (middle row), and superconducting (bottom row) phases at three different dopings. In the normal state, δ R/R ( ω , t ) is positive, with a fast decay over the whole spectrum, and independent of doping. At T =100 K, our frequency-resolved measurement reveals a more structured ω -dependence of δ R/R ( ω , t ). In under- and optimally doped samples a positive variation is measured below ∼ 1.35 eV, whereas a negative signal, with a fast decay time ( ∼ 0.5 ps), extends up to 2 eV. The temperatures, at which the high-energy negative signal appears ( T * ∼ 220 K for UD83, T * ∼ 140 K for OP96), linearly decrease as the doping increases and correspond to the onset of the universal pseudogap phase with broken time-reversal symmetry [28] . In the overdoped sample, the negative response is nearly absent, whereas the positive structure at 1.3 eV persists. Below T c , a slow δ R/R ( ω , t ) dynamics appears. This response is strongly doping-dependent, reversing sign when moving from the under- to the over-doped samples. The time-traces of the δ R/R ( ω , t ) scans at 1.5 eV probe energy ( Fig. 2 ) exactly reproduce the time-resolved reflectivities obtained in the standard single-colour configuration [29] , [30] , that is, with fixed probe wavelength. The sudden increase of the decay time in the superconducting phase is generally attributed to a bottleneck effect in which the dynamics of quasiparticles is dominated by gap-energy bosons ( ℏ Ω ∼ 2 Δ SC ) emitted during the recombination of Cooper pairs [31] , [32] , [33] . The experimental evidence of this bottleneck in a d -wave superconductor, where the nodal quasiparticles do not emit finite-energy bosons, strongly suggests that the dynamics is dominated by antinodal excitations [31] and is characterized by a transient non-thermal population in the k -space, as recently shown by time-resolved photoemission experiments [34] . These results are a benchmark for the development of realistic non-equilibrium models [6] , [35] , [36] of strongly correlated superconductors, aimed at clarifying the nature of the bosonic glue responsible for high- T c superconductivity. Figure 2: Energy- and time-resolved reflectivity on Bi 2 Sr 2 Ca 0.92 Y 0.08 Cu 2 O 8+ δ . The dynamics of the reflectivity is measured over a broad spectral range. The two-dimensional scans of δ R/R ( ω , t ) are reported for three different doping regimes (first column: underdoped (UD), T c =83 K; second column: optimally doped (OP), T c =96 K; third column: overdoped (OD), T c =86 K), in the normal (first row), pseudogap (second row) and superconducting phases (third row). See Methods for estimation of hole content p . The insets display schematically the position of each scan in the T - p phase diagram of Bi 2 Sr 2 Ca 0.92 Y 0.08 Cu 2 O 8+ δ . The white lines (right axes) are the time traces at 1.5 eV photon energy. Full size image Normal and pseudogap phases Good spectral resolution is mandatory to obtain a reliable fit of a differential dielectric function δ ɛ ( ω , t )= ɛ neq ( ω , t )− ɛ eq ( ω , t ), where ɛ neq ( ω , t ) and ɛ eq ( ω , t ) are the non-equilibrium and equilibrium dielectric functions, to the measured δ R/R ( ω , t ) ( Supplementary Note 2 ). 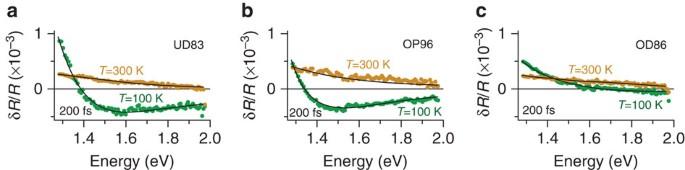Figure 3: Energy-resolved spectra and differential fit in the normal and pseudogap phases. (a–c) The maximum δR/R(ω,t)=Rneq(ω,t)/Req(ω,t)−1 (Rneq(ω,t) andReq(ω,t) being the non-equilibrium (pumped) and equilibrium (unpumped) reflectivities), measured in the normal (T=300 K, yellow dots) and pseudogap (T=100 K, green dots) phases, is reported for different doping regimes (underdoped (UD83),Tc=83 K; optimally doped (OP96),Tc=96 K; overdoped (OD86),Tc=86 K). The solid lines are the differential fit to the data. The δR/R(ω,t) related to the effective temperature increase is shown in theSupplementary Figure S2. In both the normal and the pseudogap phases, the maximum of the fast reflectivity variation is measured att=200 fs, that is, directly after all the energy of the 140 fs pump pulses has been delivered to the system. In Figure 3a,b,c we report the maximum δ R/R ( ω , t ), measured in the normal and pseudogap phases at t =200 fs. At T =300 K the fit to the data (black lines) is obtained by assuming an increase of the effective temperature, for all the doping levels. As the pseudogap phase is entered, the measured δ R/R ( ω , t ) becomes incompatible with a simple heating of the system. The nearly flat negative signal above ∼ 1.5 eV is well reproduced assuming an impulsive modification of the extended Drude model parameters, such as a weakening of the electron–boson coupling, without invoking any variation of the interband oscillators. Figure 3: Energy-resolved spectra and differential fit in the normal and pseudogap phases. ( a – c ) The maximum δ R/R ( ω , t )= R neq ( ω , t )/ R eq ( ω , t )−1 ( R neq ( ω ,t) and R eq ( ω ,t) being the non-equilibrium (pumped) and equilibrium (unpumped) reflectivities), measured in the normal ( T =300 K, yellow dots) and pseudogap ( T =100 K, green dots) phases, is reported for different doping regimes (underdoped (UD83), T c =83 K; optimally doped (OP96), T c =96 K; overdoped (OD86), T c =86 K). The solid lines are the differential fit to the data. The δ R/R ( ω , t ) related to the effective temperature increase is shown in the Supplementary Figure S2 . In both the normal and the pseudogap phases, the maximum of the fast reflectivity variation is measured at t =200 fs, that is, directly after all the energy of the 140 fs pump pulses has been delivered to the system. 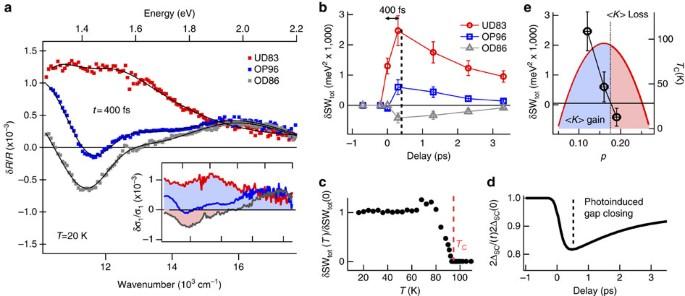Figure 4: Energy-resolved spectra and differential fit in the superconducting phase. (a) The δR/R(ω,t) att=400 fs, that is, the delay at which the maximum signal is measured, is shown for three different dopings in the superconducting phase (T=20 K). The black solid lines are differential fits to the data obtained assuming a modification of the 1.5 and 2 eV interband transitions. The values of the fitting parameters for the optimally doped sample (OP96) are reported in theSupplementary Table S2. The inset displays the relative variation of the optical conductivity for the three dopings, obtained from the data. The scale of the horizontal axis is the same as in the main panel. (b) The spectral weight variation, δSWtot=δSW1.5 eV+δSW2 eV=δω2p(1.5)/8+δω2p(2)/8 (ωp(1.5) andωp(2) being the plasma frequencies of the interband Lorentz oscillators at 1.5 and 2 eV), is reported at different delays for the three dopings. The maximum value of δSWtotcorresponds to the minimumΔSCvalue at∼400 fs, that is, after a partial electron-boson thermalization. The error bars represent the standard deviation obtained from the fit. (c) The δSWtotvalue, relative to the extrapolated zero-temperature value, is estimated from single-colour measurements and reported as a function of the temperature for OP96. Similar results are obtained for UD83 and OD86. (d) The dynamics of the superconducting gap, assuming the proportionality between δR/R(ω,t) and the photoexcited quasiparticle density21,22, is reported (Supplementary Note 4). At a pump fluence of 10 μJ cm−2, the maximum gap decrease is∼20% at 400 fs delay time. (e), The black circles represent the maximum δSWtot=δSW1.5 eV+δSW2 eV, observed at 400 fs, as a function of the doping level. The error bars take into account the stability of the differential fit on the equilibrium dielectric function (Supplementary Notes 1,2). The left axis has the same units as panelb. TheTc–pphase diagram is reported on the right-top axes. Full size image Superconducting phase In Figure 4a , we report the maximum δ R/R ( ω , t ), measured in the superconducting phase in the 1.2–2.2 eV energy range. At all doping levels, the data cannot be reproduced by modifying the extended Drude model parameters. The structured variation of the reflectivity at high energies can be only accounted for by assuming a modification of both the 1.5 and 2 eV oscillators ( Supplementary Note 2 ). The fits to the data automatically satisfy the Kramers–Kronig relations, because they are obtained as a difference between Kramers–Kronig-constrained Lorentz oscillators, and are used to calculate the relative variation of the optical conductivity (δ σ 1 / σ 1 ( ω , t ) shown in the inset of Figure 4a ). The trend from positive δ σ 1 / σ 1 ( ω , t ) in the underdoped to a slightly negative δ σ 1 / σ 1 ( ω , t ) in the overdoped samples reveals that the interband spectral weight variation (δSW tot =δ ω 2 p (1.5)/8+δ ω 2 p (2)/8, ω p (1.5) and ω p (2) being the plasma frequencies of the 1.5 and 2 eV oscillators) strongly depends on the doping. We remark that, at higher probe energies (3.14 eV), a negligible δ R/R ( t ) value for OP96 is observed, confirming that the transitions at energies larger than 2 eV are not significantly affected by the 2 Δ SC suppression. Figure 4: Energy-resolved spectra and differential fit in the superconducting phase. ( a ) The δ R/R ( ω , t ) at t =400 fs, that is, the delay at which the maximum signal is measured, is shown for three different dopings in the superconducting phase ( T =20 K). The black solid lines are differential fits to the data obtained assuming a modification of the 1.5 and 2 eV interband transitions. The values of the fitting parameters for the optimally doped sample (OP96) are reported in the Supplementary Table S2 . The inset displays the relative variation of the optical conductivity for the three dopings, obtained from the data. The scale of the horizontal axis is the same as in the main panel. ( b ) The spectral weight variation, δSW tot =δSW 1.5 eV +δSW 2 eV =δ ω 2 p (1.5)/8+δ ω 2 p (2)/8 ( ω p (1.5) and ω p (2) being the plasma frequencies of the interband Lorentz oscillators at 1.5 and 2 eV), is reported at different delays for the three dopings. The maximum value of δSW tot corresponds to the minimum Δ SC value at ∼ 400 fs, that is, after a partial electron-boson thermalization. The error bars represent the standard deviation obtained from the fit. ( c ) The δSW tot value, relative to the extrapolated zero-temperature value, is estimated from single-colour measurements and reported as a function of the temperature for OP96. Similar results are obtained for UD83 and OD86. ( d ) The dynamics of the superconducting gap, assuming the proportionality between δ R/R ( ω , t ) and the photoexcited quasiparticle density [21] , [22] , is reported ( Supplementary Note 4 ). At a pump fluence of 10 μJ cm −2 , the maximum gap decrease is ∼ 20% at 400 fs delay time. ( e ), The black circles represent the maximum δSW tot =δSW 1.5 eV +δSW 2 eV , observed at 400 fs, as a function of the doping level. The error bars take into account the stability of the differential fit on the equilibrium dielectric function ( Supplementary Notes 1,2 ). The left axis has the same units as panel b . The T c –p phase diagram is reported on the right-top axes. Full size image In the simple energy-gap model for conventional superconductors [37] , [38] , small changes of the interband transitions, over a narrow frequency range of the order of ω 0i ± Δ SC / ℏ , can arise from the opening of the superconducting gap at the Fermi level. In contrast to this model, the partial suppression of 2 Δ SC photoinduced by the pump pulse, induces a change of R ( ω , t ) over a spectral range ( ∼ 1 eV) significantly broader than 2 Δ SC ∼ 80 meV (ref. 39 ). This result reveals a dramatic superconductivity-induced modification of the Cu–O electronic excitations at 1.5 and 2 eV. In the time-domain, we obtain that the dynamics of δSW tot (reported in Fig. 4b ) is nearly exponential with a time constant ô =2.5±0.5 ps. The δSW tot variation is completely washed out at longer times (>5 ps), when the complete electron–boson thermalization broadens the Drude peak, overwhelming the contribution of δSW tot . It is worth noting that the photoinduced modifications of δSW tot vanish as T c is approached from below ( Fig. 4c ), demonstrating that this effect is exclusively related to the impulsive partial suppression of 2 Δ SC . Further evidence of the direct relation between 2 Δ SC and δSW tot is obtained from a comparison with time-resolved experiments with probe energy in the mid-infrared [40] and THz regions [41] , [42] , directly showing a recovery time of the superconducting gap and condensate ranging from 2 to 8 ps, for different families of cuprates and different experimental conditions (that is, temperature and pump fluence). The correspondence between these timescales and the recovery time of δSW tot finally demonstrates the interplay between the excitations at 1.5 and 2 eV and the superconducting gap 2 Δ SC . In addition, our results clarify the origin of the doping- and temperature-dependent δ R/R ( t ) signal measured in single-colour experiments [24] , [29] , [30] , [31] , [32] , [33] at high-energy scales and demonstrate that the dynamics of 2 Δ SC ( t ) can be reconstructed exploiting the δ R/R ( t ) signal measured at high-energies ( Fig. 4d and Supplementary Note 4 ). Assuming that the total spectral weight change of the interband transitions is compensated by an opposite change of the Drude-like optical conductivity, we can estimate a superconductivity-induced kinetic energy decrease of ∼ 1–2 meV per Cu atom for the underdoped sample (Methods). This value is very close to the superconductivity-induced kinetic energy gain predicted by several unconventional models [43] , [44] . As we move from the under- to the over-doped side of the superconducting dome ( Fig. 4e ), we obtain that the modification of the SW of optical transitions, involving excitations at 1.5 and 2 eV, completely accounts for the transition from a superconductivity-induced gain to a loss of kinetic energy [12] , [17] , [18] , [19] , [20] , estimated by equilibrium optical spectroscopies, directly measuring the low-energy optical properties, and single-colour time-resolved reflectivity measurements [29] . This result indicates that most of the superconductivity-induced modifications of the excitation spectrum and optical properties at the low-energy scale are compensated by a variation of the in-plane electronic excitations at 1.5 and 2 eV, demonstrating that these excitations are at the base of an unconventional superconductive mechanism both in the under- and over-doped sides of the superconducting dome. In conclusion, we have exploited the time-resolution of a novel pump-supercontinuum-probe optical spectroscopy to unambiguously demonstrate that, in Bi 2 Sr 2 Ca 0.92 Y 0.08 Cu 2 O 8+ δ , the superconductive transition is strongly unconventional both in the under- and over-doped sides of the superconducting dome, involving in-plane Cu–O excitations at 1.5 and 2 eV. When moving from below to above the optimal hole doping, the spectral weight variation of these features entirely accounts for a crossover from a superconductivity-induced gain to a BCS-like loss of the carrier kinetic energy [4] , [19] , [20] . Superconductivity-induced changes of the optical properties at high-energy scales ( ℏ ω >100 Δ SC ) seem to be a universal feature of high-temperature superconductors [5] , [7] , [11] , indicating that the comprehension of the interplay between low-energy excitations and the high-energy scale physics, associated with Mott-like excitations, will be decisive in understanding high-temperature superconductivity. Pump-supercontinuum-probe technique The optical pump-probe setup is based on a cavity-dumped Ti:sapphire oscillator. The output is a train of 800 nm–140 fs pulses with an energy of 40 nJ per pulse. A 12-cm-long photonic crystal fibre, with a 1.6-μm core, is seeded with 5 nJ per pulse focused onto the core by an aspherical lens. The supercontinuum probe output is collimated and refocused on the sample through achromatic doublets in the near-IR/visible range. The 800 nm oscillator output (pump) and the supercontinuum beam (probe), orthogonally polarized, are non-collinearly focused onto the sample. The superposition on the sample and the spot dimensions (40 μm for the IR-pump and 20 μm for the supercontinuum probe) are monitored through a charge-coupled device camera. The pump fluence is ∼ 10 μJ cm −2 . The probe beam impinges on the sample surface nearly perpendicularly, ensuring that the ab -plane reflectivity is measured. The reflected probe beam is spectrally dispersed through an SF11 equilateral prism and imaged on a 128-pixel-linear photodiode array (PDA), capturing the 620–1,000 nm spectral region. A spectral slice, whose width ranges from 2 at 620 nm to 6 at 1,000 nm, is acquired by each pixel of the array. The probe beam is sampled before the interaction with the pump and used as a reference for the supercontinuum intensity. The outputs of the two PDAs are acquired through a 22 bit/2 MHz fast digitizer, and are divided pixel by pixel to compensate the supercontinuum intensity fluctuations, obtaining a signal to noise ratio of the order of 10 −4 acquiring 2,000 spectra in about 1 s. The differential reflectivity signal is obtained modulating the pump beam with a mechanical chopper and performing the difference between unpumped and pumped spectra. The spectral and temporal structure of the supercontinuum pulse has been determined either by exploiting the switching character of the photo-induced insulator-to-metal phase transition in a VO 2 multifilm [23] or by standard XFROG techniques. The data reported in Figure 2 have been corrected taking into account the spectral and temporal structure of the supercontinuum pulse. Spectroscopic ellipsometry The ab -plane dielectric function of the Bi 2 Sr 2 Ca 0.92 Y 0.08 Cu 2 O 8+ δ samples has been obtained by applying the Kramers–Kronig relations to the reflectivity for 50 cm −1 < ω /2πc<6,000 cm −1 and directly from ellipsometry for 1,500 cm −1 < ω /2π c <36,000 cm −1 . This combination allows a very accurate determination of ɛ ( ω ) in the entire combined frequency range. Due to the off-normal angle of incidence used with ellipsometry, the ab -plane pseudo-dielectric function had to be corrected for the c -axis admixture. Samples The Y-substituted Bi2212 single crystals were grown in an image furnace by the travelling-solvent floating-zone technique with a non-zero Y content in order to maximize T c (ref. 45 ). The underdoped samples were annealed at 550 °C for 12 days in a vacuum-sealed glass ampoule with copper metal inside. The overdoped samples were annealed in a quartz test tube under pure oxygen flow at 500 °C for 7 days. To avoid damage of the surfaces, the crystals were embedded in Bi 2 Sr 2 CaCu 2 O 8+ δ powder during the annealing procedure. In both cases, the quartz tube was quenched to ice-water bath after annealing to preserve the oxygen content at annealing temperature. For the optimally doped sample (OP96), the critical temperature reported ( T c =96 K) is the onset temperature of the superconducting phase transition, the transition being very narrow (Δ T c <2 K). As a meaningful parameter for the under- ( T c =83 K, UD83) and over-doped ( T c =86 K, OD86) samples, which have respective transition widths of Δ T c ∼ 8 K and Δ T c ∼ 5 K, we report the transition midpoint temperatures. The hole concentration p is estimated through the phenomenological formula [46] T c / T c,max =1–82.6·( p −0.16) 2 , where T c,max is the critical temperature of the optimally doped sample. Kinetic energy Below the critical temperature T c , possible modifications of the high-energy spectral weight , including the contribution to the optical conductivity from all the possible interband transitions i , must compensate the spectral weight of the condensate zero-frequency δ -function, SW δ , and the variation of the spectral weight of the Drude-like optical conductivity, , related to the free carriers in the conduction band. This is expressed by the Ferrell–Glover–Tinkham sum rule [4] : where the superscripts refer to the normal (N) and superconducting (SC) phases. In the special case of a single conduction band within the nearest-neighbour tight-binding model [43] , [44] , the total intraband spectral weight SW D can be related to the kinetic energy T δ of the charge carriers (holes) associated to hopping process in the δ direction, via the relation [43] : where a δ is the lattice spacing in the Cu–O plane, projected along the direction determined by the in-plane polarization δ of the incident light and V Cu is the volume per Cu atom. We obtain 〈 K 〉=2〈 T δ 〉 from the spectral weight variation of the interband oscillators, through the relation: Considering V Cu =V unit cell /8 ∼ 1.1·10 −22 cm 3 and a δ =a unit cell /√2 ∼ 3.9 Å, we obtain that the kinetic energy can be calculated as 〈 K 〉 =8 ℏ 2 [SW h N –SW h SC ]·(83 meV/eV 2 ), where 8 ℏ 2 [SW h N –SW h SC ] is the interband spectral weight variation expressed in eV 2 . A finite value of SW h N –SW h SC thus implies a superconductivity-induced variation of the kinetic energy. To obtain the total kinetic energy variation related to the condensate formation, we estimate a photo-induced breaking of ∼ 3–7% of the Cooper pairs ( Supplementary Note 3 ), and we extrapolate the measured SW h N –SW h SC values, reported in Figure 4c–e , to the values corresponding to the breaking of 100% of the Cooper pairs. How to cite this article: Giannetti, C. et al . Revealing the high-energy electronic excitations underlying the onset of high-temperature superconductivity in cuprates. Nat. Commun. 2:353 doi: 10.1038/ncomms1354 (2011).